Green synthesis of nitriles using non-noble metal oxides-based nanocatalysts (Hetero)aromatic and aliphatic nitriles constitute major building blocks for organic synthesis and represent a versatile motif found in numerous medicinally and biologically important compounds. In general, these nitriles are synthesized by traditional cyanation procedures using toxic cyanides. With respect to green chemistry, the development of more sustainable and cost-efficient processes for the synthesis of advanced nitriles is highly desired. Here we report an environmentally benign synthesis of all kinds of structurally diverse aryl, heterocyclic, allylic and aliphatic nitriles from easily available alcohols applying aqueous ammonia and molecular oxygen. Key to success for this synthesis is the use of nitrogen-doped graphene-layered non-noble metal oxides as stable and durable nanocatalysts. As an example a renewable synthesis of adiponitrile, an industrially important bulk chemical is presented. Organic nitriles have an important role as integral part of pharmaceuticals, agrochemicals and fine chemicals. In fact in 2010, more than 30 pharmaceuticals bearing cyano groups were prescribed for diverse medicinal indications and >20 additional nitrile-containing compounds were in clinical development [1] , [2] . Besides, they serve as common building blocks for high performance materials, polymers and molecular electronics [2] , [3] , [4] . In organic chemistry, nitriles serve as essential intermediates for the production of a variety of heterocycles [5] , [6] , as well as precursors for amines, amides, aldehydes and different carboxylic acid derivatives [7] , [8] . For their synthesis, commonly highly toxic HCN or metal cyanides (for example, HCN: TD Lo =0.055 mg kg −1 (human, intravenous); KCN: LD 50 =5–10 mg kg −1 (oral in rats, mice, rabbits); Zn(CN) 2 : LD 50 =54 mg kg −1 (oral in rats)) have to be applied for nucleophilic substitutions of alkyl and aryl halides [9] , [10] or the classic Sandmeyer reaction [11] . Apart from the toxicity, which led to one of the worst environmental disasters in Europe (cyanide spill in Baia Mare, Romania, 2000), the use of metal cyanides generates significant amount of waste. Today in the chemical industry, ammoxidation is the preferred method to produce acrylonitrile, methacrylonitrile, aryl nitriles (limited to simple benzonitriles) and heteroaromatic nitriles (limited to cyanopyridines and pyrazine nitriles) on a bulk-scale [12] , [13] , [14] , [15] . However, most of these processes are performed under drastic conditions and consequently they are restricted to non-functionalized substrates. In fact, no general ammoxidation reaction exists so far, which allows for the synthesis of a broad range of functionalized nitriles including more valuable heterocycles. Hence, there is a general need for alternative and sustainable routes for –CN introduction in structurally diverse molecules. In this respect, the use of alcohols as starting materials [16] , [17] , [18] , [19] , [20] , [21] , [22] is highly desired, as they are easily accessible and of increasing importance as renewable feedstock [16] , [17] , [18] , [19] , [20] , [21] , [22] . Key to success for such reactions is the development of suitable, selective and cost-effective catalyst systems. In the past, heterogeneous ruthenium [22] and homogeneous copper-based catalysts [23] , [24] , [25] , [26] , [27] have been used for the conversion of alcohols and amines to the corresponding nitriles. Despite these developments, still practical, and easily re-usable, as well as cost-efficient heterogeneous catalysts are highly desired for the synthesis of advanced nitriles from alcohols. In the last decade, the development of non-noble metal-based catalysts [28] , [29] , [30] , [31] , especially nanomaterials [32] , [33] , [34] , for organic synthesis has become a prime topic and is crucial for the advancement of green and sustainable industrial processes. Last year, we reported the preparation of nanoscale cobalt and iron oxides, which constitute excellent catalysts for highly selective hydrogenation process [33] , [34] . We also showed that pyrolysis of metal acetate-nitrogen ligated complexes on carbon leads to the formation of nanoscale metal oxides (Co 3 O 4 -NGr/C; Fe 2 O 3 -NGr/C), which are surrounded by nitrogen-doped graphene layers (NGr). In the present work, we demonstrate the selectivity of such non-noble metal oxides-based nanocatalysts (Co 3 O 4 -NGr/C; Fe 2 O 3 -NGr/C) activated by nitrogen-doped graphene surfaces in challenging oxidation reactions for the synthesis of all kinds of aromatic, heterocyclic and aliphatic nitriles from alcohols and aqueous (aq.) ammonia using molecular oxygen. 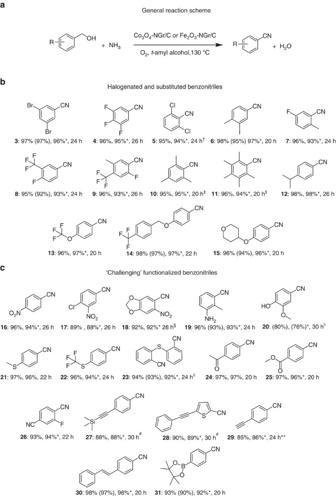Figure 1:Synthesisof substituted and functionalized benzonitriles. (a) General reaction scheme. (b) Halogeneted and substituted benzonitriles. (c) ‘Challenging’ functionalyzed benzonzonitriles. Reaction conditions: 0.5 mmol alcohol, 40 mg Co3O4-NGr/C (4 mol% Co), 100 μl aq. NH3, 5 bar O2, 4 mlt-amyl alcohol, 130 °C. Conversions, yields and products were determined by GC (using 100 μLn-hexadecane as standard) and GC–MS analysis. * with 45 mg Fe2O3-NGr/C (4.5 mol% Fe). † with 6 mol% catalyst at 150 °C. ‡in 4 ml H2O. § with 5-6 mol% catalyst at 140 °C. || 300 μl aq. NH3. # with 6 mol% catalyst. ** in 1:1t-amyl alcohol-H2O from 4-(trimethylsilylethynyl)benzyl alcohol. Yields in parentheses refer to isolated yields using Co3O4-NGr/C catalyst. Preparation and activity of metal oxide-based nanocatalysts A series of non-noble metal-based catalysts was prepared by pyrolysis of the respective metal acetate-phenanthroline complexes on Vulcan at 800 °C under argon (see Supplementary Methods , Supplementary Figs 1–11 ; and Supplementary Table 1 for detailed characterization). All these materials were tested for their catalytic activity for the benchmark oxidation of benzyl alcohol to benzonitrile. As seen from Table 1 , defined metal complexes as well as carbon supported non-pyrolyzed materials showed little activity ( Table 1 , entries 1–21). Similarly, pyrolyzed metal salts on carbon without any phenanthroline ligand present gave only slight conversion ( Table 1 , entries 22–28). Notably, pyrolysis of metal-phenanthroline complexes showed varying catalytic activities ( Table 1 entries, 29–35). The pyrolyzed cobalt-phenanthroline (Co 3 O 4 -NGr/C) and iron-phenanthroline (Fe 2 O 3 -NGr/C) based materials are found to be excellent catalysts producing benzonitrile in nearly quantitative yield (98%; Table 1 , entries 29–30). The copper-based catalyst exhibited moderate activity (54% yield; Table 1 , entry 31), whereas the other catalysts based on Mn, Cr, V and Ni showed only poor activity ( Table 1 , entries 32–35). To demonstrate the recycling of the catalyst, Co 3 O 4 -NGr/C was used for the benchmark reaction. Up to four times the catalyst can be easily used without re-activation (see Methods section). Table 1 Synthesis of benzonitrile using different catalysts. Full size table Applying cobalt (Co 3 O 4 -NGr/C; Co-phenanthroline/C-800) and iron (Fe 2 O 3 -NGr/C; Fe-phenanthroline/C-800) oxide-based catalysts, we demonstrated the general synthesis of nitriles from corresponding alcohols in liquid phase. Synthesis of substituted and functionalized benzonitriles Benzonitriles, which are substructures of different products of our daily lives, have been obtained in good to excellent yields ( Figs 1 and 2 ). Interesting halogenated benzonitriles were prepared in 93–97% yields. For example, 2,6-dichlorobenzonitrile, which is a herbicide and a key intermediate for the preparation of a series of highly potential pesticides and various special kinds of engineering plastics, has been synthesized in 94–95% yields ( Fig. 1 ). Sterically hindered tri- and penta-methyl substituted substrates, which do not undergo selective ammoxidation were completely converted to the corresponding benzonitriles in 94–96% yields. Furthermore, –NO 2 , –NH 2 and –OH substituted benzonitriles, which are difficult to access by ammoxidation [12] have been selectively obtained in up to 96% yields ( Fig. 1 ). To our delight, even sensitive functional groups such as thio-ether, amide, sulphide, ketone, C–C double and triple bonds, as well as C–Si and C–B bonds are well tolerated. Figure 1: Synthesis of substituted and functionalized benzonitriles. ( a ) General reaction scheme. ( b ) Halogeneted and substituted benzonitriles. ( c ) ‘Challenging’ functionalyzed benzonzonitriles. Reaction conditions: 0.5 mmol alcohol, 40 mg Co 3 O 4 -NGr/C (4 mol% Co), 100 μl aq. NH 3 , 5 bar O 2 , 4 ml t -amyl alcohol, 130 °C. Conversions, yields and products were determined by GC (using 100 μL n -hexadecane as standard) and GC–MS analysis. * with 45 mg Fe 2 O 3 -NGr/C (4.5 mol% Fe). † with 6 mol% catalyst at 150 °C. ‡in 4 ml H 2 O. § with 5-6 mol% catalyst at 140 °C. || 300 μl aq. NH 3 . # with 6 mol% catalyst. ** in 1:1 t -amyl alcohol-H 2 O from 4-(trimethylsilylethynyl)benzyl alcohol. Yields in parentheses refer to isolated yields using Co 3 O 4 -NGr/C catalyst. 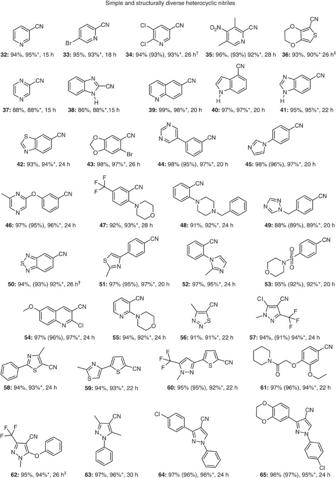Figure 2: Synthesis of structurally diverse heterocyclic nitriles. Reaction conditions: 0.5 mmol alcohol, 40 mg Co3O4-NGr/C (4 mol% Co), 100 μl aq. NH3, 5 bar O2, 4 mlt-amyl alcohol, 130 °C. Conversions, yields and products were determined by GC (using 100 μln-hexadecane as standard) and GC–MS analysis. * with 45 mg Fe2O3-NGr/C (4.5 mol% Fe). † at 140oC. ‡ with 60 mg catalyst (6 mol%). Yields in parentheses refer to isolated yields using Co3O4-NGr/C catalyst. Full size image Figure 2: Synthesis of structurally diverse heterocyclic nitriles. Reaction conditions: 0.5 mmol alcohol, 40 mg Co 3 O 4 -NGr/C (4 mol% Co), 100 μl aq. NH 3 , 5 bar O 2 , 4 ml t -amyl alcohol, 130 °C. Conversions, yields and products were determined by GC (using 100 μl n -hexadecane as standard) and GC–MS analysis. * with 45 mg Fe 2 O 3 -NGr/C (4.5 mol% Fe). † at 140 o C. ‡ with 60 mg catalyst (6 mol%). Yields in parentheses refer to isolated yields using Co 3 O 4 -NGr/C catalyst. Full size image Synthesis of heterocyclic nitriles Cyano-substituted heterocycles are important substructures in many medicinal compounds. In general, these products are synthesized by cyanation from the corresponding heteroaryl halides [9] , [10] . Advantageously, applying our methodology a broad series of heterocyclic nitriles along with aryl nitriles bearing heterocyclic backbones were synthesized in good to excellent yields ( Fig. 2 ). Synthesis of allylic and aliphatic nitriles Compared with the ammoxidation towards aromatic nitriles, the synthesis of allylic and aliphatic nitriles has been much less studied [12] . Therefore, we were interested in the performance of our catalysts with such substrates. As shown in Fig. 3 , all the tested allylic alcohols have been selectively oxidized to give the corresponding nitriles in up to 93% yields. In these cases no significant oxidation of the olefinic bond took place. Next, the oxidation of various aliphatic alcohols was performed. To get sufficient reactivity, the reaction temperature had to be increased under different reaction conditions. Nevertheless, 15 different aliphatic nitriles were obtained in up to 82% yields ( Fig. 3 ). 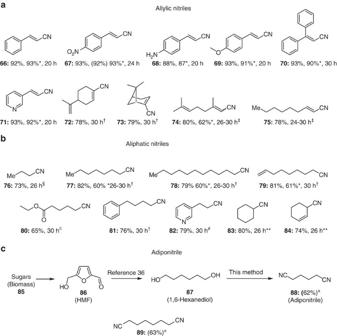Figure 3: Synthesis of allylic and aliphatic nitriles. (a) Allylic nitriles. (b) Aliphatic nitriles. (c) Adiponitrile. Reaction conditions: 0.5 mmol alcohol, 40 mg Co3O4-NGr/C (4 mol% Co), 100 μl aq. NH3, 5 bar O2, 4 mlt-amyl alcohol, 130 °C. * with 45 mg Fe2O3-NGr/C (4.5 mol% Fe). † 1 mmol alcohol, 5 mol% Co3O4-NGr/C (*6 mol% Fe2O3-NGr/C), 300 μl aq. NH3, 2:1 (or 3:1) water-n-heptane (6 ml), 140 °C, 5 bar O2. ‡ 1 mmol alcohol, 5 mol% Co3O4-NGr/C (*6 mol% Fe2O3-NGr/C), 300 μl aq. NH3, 1:1 water-n-heptane (6 ml), 140 °C, 5 bar O2. § 2 mmol alcohol, 5 mol% Co3O4-NGr/C, 600 μl aq. NH3,2:1 water:t-butanol, 130 °C, 5 bar O2. || 1 mmol alcohol, 5 mol% Co3O4-NGr/C catalyst, 300 μl aq. NH3,t-amyl alcohol 150 °C, 5 bar O2. #1 mmol alcohol, 5 mol% Co3O4-NGr/C catalyst, 300 μl aq. NH3,t-amyl alcohol ort-butanol, 150 °C, 5 bar O2. **1 mmol alcohol, 5 mol% Co3O4-NGr/C catalyst, 300 μl aq. NH3, 6 ml water, 140 °C.±1 mmol diol, 25 mol% K2CO3and weight of Co3O4-NGr/C-catalyst corresponds to 4 mol% Co for each –CH2-OH conversion, 600 μl aq. NH3,8 mlt-amyl alcohol, 150 °C, 48 h, 5 bar O2, isolated yields. Conversions, yields and products were determined by GC (usingn-hexadecane as standard) and GC–MS analysis. Yields in parentheses refer to isolated yields using Co3O4-NGr/C catalyst. Figure 3: Synthesis of allylic and aliphatic nitriles. ( a ) Allylic nitriles. ( b ) Aliphatic nitriles. ( c ) Adiponitrile. Reaction conditions: 0.5 mmol alcohol, 40 mg Co 3 O 4 -NGr/C (4 mol% Co), 100 μl aq. NH 3 , 5 bar O 2 , 4 ml t -amyl alcohol, 130 °C. * with 45 mg Fe 2 O 3 -NGr/C (4.5 mol% Fe). † 1 mmol alcohol, 5 mol% Co 3 O 4 -NGr/C (*6 mol% Fe 2 O 3 -NGr/C), 300 μl aq. NH 3 , 2:1 (or 3:1) water- n -heptane (6 ml), 140 °C, 5 bar O 2 . ‡ 1 mmol alcohol, 5 mol% Co 3 O 4 -NGr/C (*6 mol% Fe 2 O 3 -NGr/C), 300 μl aq. NH 3 , 1:1 water- n -heptane (6 ml), 140 °C, 5 bar O 2 . § 2 mmol alcohol, 5 mol% Co 3 O 4 -NGr/C, 600 μl aq. NH 3, 2:1 water: t -butanol, 130 °C, 5 bar O 2 . || 1 mmol alcohol, 5 mol% Co 3 O 4 -NGr/C catalyst, 300 μl aq. NH 3, t -amyl alcohol 150 °C, 5 bar O 2 . #1 mmol alcohol, 5 mol% Co 3 O 4 -NGr/C catalyst, 300 μl aq. NH 3 , t -amyl alcohol or t -butanol, 150 °C, 5 bar O 2 . **1 mmol alcohol, 5 mol% Co 3 O 4 -NGr/C catalyst, 300 μl aq. NH 3 , 6 ml water, 140 °C.±1 mmol diol, 25 mol% K 2 CO 3 and weight of Co 3 O 4 -NGr/C-catalyst corresponds to 4 mol% Co for each –CH 2 -OH conversion, 600 μl aq. NH 3, 8 ml t -amyl alcohol, 150 °C, 48 h, 5 bar O 2 , isolated yields. Conversions, yields and products were determined by GC (using n -hexadecane as standard) and GC–MS analysis. Yields in parentheses refer to isolated yields using Co 3 O 4 -NGr/C catalyst. Full size image Further, we developed a sustainable synthesis for industrially important adiponitrile. This dinitrile is used for the manufacture of the common polymer nylon 6,6. In 2005, the global production of adiponitrile reached more than 1.5 million tons per annum [35] . The current industrial process is based on the Ni-catalysed hydrocyanation of 1,3-butadiene. In our novel process, the desired product is obtained by selective oxidation of 1,6-hexanediol which can be derived from biomass [36] as shown in Fig. 3 , in the presence of aq. ammonia and molecular oxygen ( Fig. 3 ). Finally, to demonstrate the synthetic utility of this novel method, we performed the ammoxidation of several benzyl alcohols on a 5-g scale. For all the tested substrates, similar yields to the 0.5-mmol scale were obtained ( Fig. 4 ). 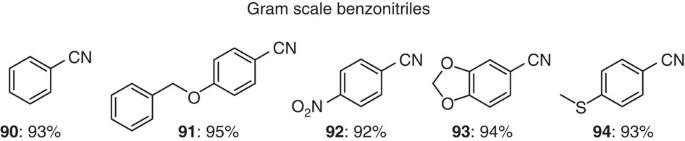Figure 4: Gram scale reactions. Reaction conditions: 5 g alcohol, weight of Co3O4-NGr/C catalyst corresponds to 4 mol% Co, 100 μl aq. NH3for each 0.5 mmol substrate, 130 °C, 100–150 mlt-amyl alcohol, 20–30 h. Isolated yields. Figure 4: Gram scale reactions. Reaction conditions: 5 g alcohol, weight of Co 3 O 4 -NGr/C catalyst corresponds to 4 mol% Co, 100 μl aq. NH 3 for each 0.5 mmol substrate, 130 °C, 100–150 ml t -amyl alcohol, 20–30 h. Isolated yields. Full size image Based on the results vide supra , we propose the following general reaction pathway for the synthesis of nitriles from alcohols catalysed by cobalt and iron oxide-based nanomaterials using molecular oxygen and aq. ammonia ( Fig. 5 ). Initially, catalytic aerobic oxidation of alcohol to the corresponding aldehyde is observed. In most cases the respective aldehyde can be determined during the progress of the reaction. Next, the aldehyde undergoes condensation with ammonia and forms the corresponding imine. Notably, this imine is unstable and is immediately oxidized to give nitrile as the final product. In this reaction sequence, water is produced as the only by-product. 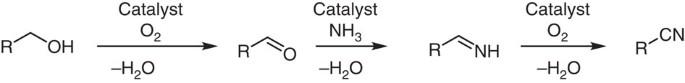Figure 5: General reaction pathway for the synthesis of nitriles from alcohols. R=aromatic; aliphatic; heterocyclic; allylic. Figure 5: General reaction pathway for the synthesis of nitriles from alcohols. R=aromatic; aliphatic; heterocyclic; allylic. Full size image In summary, we developed a general green process for the synthesis of nitriles from easily accessible alcohols applying cheap and abundant reagents such as molecular oxygen and aq. ammonia. Key to success for this achievement is the use of stable, durable and cost-efficient cobalt or iron oxide-based nanocatalysts. Noteworthy, structurally demanding and functionalized benzonitriles, which are difficult to prepare by classical ammoxidation or cyanation processes were synthesized in good to excellent yields. The high synthetic utility of this method is also demonstrated in the synthesis of structurally diverse heterocyclic nitriles, which represent important building blocks for life science applications. The more challenging allylic and aliphatic alcohols have been selectively converted into corresponding nitriles too. Using our protocol, we obtained adiponitrile, which is an important feedstock for the nylon 6,6 polymer, from renewable feedstock. The catalyst was successfully recycled and reused without significant deactivation. The use of more abundant non-noble metal-based catalysts, molecular oxygen, aq. ammonia and alcohols as starting materials made this process simple, economical and sustainable. Materials and general analytical methods Alcohols, metal precursors, aq. ammonia (320145 ACS reagent, 28.0–30.0% NH 3 basis, Sigma-Aldrich) and other chemicals were obtained from various chemical companies. Carbon powder, VULCAN XC72R with Code XVC72R and CAS No. 1333-86-4 was obtained from Cabot Corporation Prod. The pyrolysis experiments were carried out in Nytech-Qex oven. 5-(2-Phenyleth-1-ynyl)thiophene-2-methanol and β-Phenylcinnamyl alcohol were prepared from the corresponding aldehydes. Transmission electron microscopy measurements were performed at 200 kV with an aberration-corrected JEM-ARM200F (JEOL, Corrector: CEOS). The microscope is equipped with a JED-2300 (JEOL) energy-dispersive X-ray-spectrometer for chemical analysis. The samples were deposited without any pretreatment on a holey carbon supported Cu-grid (mesh 300) and transferred to the microscope. The high-angle annular dark field and annular bright field images were recorded with a spot size of ~0.1 nm, a probe current of 120 pA and a convergence angle of 30–36°. The collection semi-angles for high-angle annular dark field and annular bright field were 70–170 mrad and 11–22 mrad, respectively. XPS (X-ray Photoelectron Spectroscopy) data were obtained with a VG ESCALAB220iXL (ThermoScientific) with monochromatic Al Kα (1,486.6 eV) radiation. The electron binding energies E B were obtained without charge compensation. For quantitative analysis the peaks were deconvoluted with Gaussian–Lorentzian curves, the peak area was divided by a sensitivity factor obtained from the element specific Scofield factor and the transmission function of the spectrometer. EPR (Electron Paramagnetic Resonance) spectra in X-band were recorded on a Bruker EMX CW-micro spectrometer equipped with an ER 4119HS-WI high-sensitivity cavity and a variable temperature control unit using the following parameters: microwave power=6.64 mW, modulation frequency=100 kHz, modulation amplitude=1 G. Mössbauer spectra were obtained at 300 K and 77 K by a Mössbauer spectrometer from Wissel GmbH equipped with a 57 Co source. Isomer shifts are given relative to α-Fe at room temperature. The spectra were analysed by least-square fits using Lorentzian line shapes. GC (gas chromatography) conversions and yields were determined by GC-FID, HP6890 with FID detector, column HP530 m × 250 mm × 0.25 μm. NMR (nuclear magnetic resonace) data were recorded on a Bruker ARX 300 and Bruker ARX 400 spectrometers. All catalytic experiments were carried out in 300 ml and 100 ml autoclaves (PARR Instrument Company). To avoid unspecific reactions, all catalytic reactions were carried out either in glass vials which were placed inside the autoclave or Teflon vessel-fitted autoclaves. Procedure for the preparation of catalysts The following metal salts were used for the preparation of catalysts: Co(OAc) 2 .4H 2 O, Fe(OAc) 2 , Ni(OAc) 2 .4H 2 O, Cu(OAc) 2 .H 2 O, Mn(OAc) 2 .4H 2 O, V(acac) 3 and Cr(acac) 3 . A mixture of respective metal salt (corresponds to 3 wt%) and 1,10-phenanthroline (metal:phenanthroline=1:2 mole ratio; in case of iron Fe: phenanthrolin=1:3) in ethanol was stirred for 30–40 min at room temperature. Then, vulcan XC72R carbon powder was added and the whole reaction mixture was stirred at 60 °C for 5–6 h (15 h in case of iron). The reaction mixture was cooled to room temperature and ethanol was removed slowely under vacuum. The remaining solid sample obtained was dried at 60 °C for 12 h. The dried sample was ground to a powder. Then, the powdered sample was pyrolyzed at 800 °C for 2 h in argon atmosphere and cooled to room temperature. Elemental analysis of Co-phenanthroline/C (Wt%): C=89.68, H=0.199, N=2.70, Co=3.05. Elemental analysis of Fe-phenanthroline/C (wt%): C=91.1, H=0.19, N=2.69, Fe=2.95. General procedure for the synthesis of nitriles The magnetic stirring bar and corresponding alcohol were transferred to the glass vial and then solvent was added. The catalyst was added followed by the addition of aq. NH 3 . Then the vial was fitted with septum, cap and needle. The reaction vials were placed into an autoclave and the autoclave was pressurized to 5 bar molecular oxygen. Reactions were also carried out directly in the Teflon-fitted autoclaves wherever required. The autoclave was placed into heating system and temperature controller (placed 30 min before counting the reaction time to attain reaction temperature). The temperature of the heating system is set to get the exact desired temperature inside the autoclave and the temperature measured inside the autoclave was taken as the reaction temperature (in case of autoclave placed in the aluminium block heating system, the temperature of the aluminium block was set to get the required reaction temperature inside the autoclave. Temperature of the aluminium block was set at 10–12 °C more to get the perfect reaction temperature inside the autoclave). The reaction was stirred for required time and after the completion of the reaction, the autoclave was cooled to room temperature. The remaining oxygen was discharged and the samples were removed from the autoclave. To the individual vials, n -hexadecane as standard was added and the reaction product was diluted with ethyl acetate followed by filtration and then analysed by GC and GC mass spectrometry (GC–MS). Qualitative and quantitative analysis of all products were made using GC and GC–MS analysis. In case of reactions run in water, for aromatic substrates the catalyst was filtered off and washed with ethyl acetate and then reaction products were extracted with ethyl acetate. The ethyl acetate extract was concentrated and then n -hexadecane was added and subjected to GC analysis. Except for butyl nitrile, in case of reactions run in water and water-organic solvent mixtures, catalyst was filtered off, washed with tetrahydrofuran (THF) and solvent was removed. Finally diluted with ethyl acetate or THF followed by the addition of n -hexadecane and subjected to GC and GC–MS analysis. In case of butyl nitrile, the reaction products were diluted with THF, catalyst was filtered off and subjected to GC and GC–MS. For synthesis of dinitriles, the reaction of diols was carried out under the experimental condition mentioned in Fig. 3 in one step for 48 h. In an alternative procedure, the reaction of diol was carried out for 24 h under the reaction conditions mentioned in Fig. 3 and then the crude product mixture was isolated. In the next step the reaction of isolated crude product was continued for another 24 h under similar experimental conditions by adding fresh catalyst, solvent, base and aq. ammonia. Procedure for products isolation Under similar experimental conditions vide supra , after completion of the reaction, the autoclave was cooled to room temperature. The remaining oxygen was discharged and the sample was removed from the autoclave. Catalyst from the reaction mixture was filtered off and washed with ethyl acetate. The solvent from filtrate containing reaction product was removed in vacuo. The corresponding nitrile was purified by column chromatography (silica; n -hexane-ethyl acetate mixture). Then, dried over anhydrous Na 2 SO 4 and the solvent was removed in vacuo followed by drying. Products were analysed and characterized by GC, GC–MS and NMR ( Supplementary Figs 12–55 ) spectral analysis. Procedure for catalyst recycling The recycling of catalyst experiments was carried out using benzyl alcohol, as model substrate applying standard procedure under following reaction conditions: 1 mmol benzyl alcohol, 80 mg Co 3 O 4 -NGr/C, 200 μl aq. NH 3 , 130 °C, 15–24 h, 5 bar O 2 , 8 ml t -amyl alcohol. After completion of the reaction, in each run the catalyst was separated by centrifugation, washed with ethyl acetate and dried. The dried catalyst was used for the next run without re-activation. Alternatively, after completion of the reaction, the reaction solution was carefully decanted and the fresh solvent, substrate and ammonia were added and the reaction was performed. Conversion and yield were determined by GC analysis using n -hexadecane as standard. The catalyst can be used up to four times without any re-activation, with benzonitrile yields of 98%, 97%, 96% and 92% obtained after 0, 1, 2, and 3 rounds of recycling respectively. Procedure for gram scale reactions To a Teflon-fitted 300-ml autoclave, the magnetic stirring bar and corresponding alcohol were transferred and then solvent was added. The catalyst (Co 3 O 4 -NGr/C-800) was added followed by the addition of aq. NH 3 . The autoclave was pressurized to 5 bar molecular oxygen. The autoclave was placed into an aluminium block (placed 30 min before counting the reaction time to attain reaction temperature) and the temperature of the aluminium block was set to get the required reaction temperature inside the autoclave. The reactions were stirred for required time and after the completion of the reaction, the autoclave was cooled to room temperature. The remaining oxygen was discharged and the samples were removed from the autoclave. The catalyst was filtered off and washed with ethyl acetate. The solvent from the filtrate containing reaction product was removed and diluted with ethyl acetate. The corresponding nitriles was purified by column chromatography, (silica; n -hexane-ethyl acetate mixture) dried over anhydrous Na 2 SO 4 , and solvent was removed and dried finally. How to cite this article: Jagadeesh, R. V. et al. Green synthesis of nitriles using non-noble metal oxides-based nanocatalysts. Nat. Commun. 5:4123 doi: 10.1038/ncomms5123 (2014).